Targeted delivery of colloids by swimming bacteria The possibility of exploiting motile microorganisms as tiny propellers represents a fascinating strategy for the transport of colloidal cargoes. However, delivery on target sites usually requires external control fields to steer propellers and trigger cargo release. The need for a constant feedback mechanism prevents the design of compact devices where biopropellers could perform their tasks autonomously. Here we show that properly designed three-dimensional (3D) microstructures can define accumulation areas where bacteria spontaneously and efficiently store colloidal beads. The process is stochastic in nature and results from the rectifying action of an asymmetric energy landscape over the fluctuating forces arising from collisions with swimming bacteria. As a result, the concentration of colloids over target areas can be strongly increased or depleted according to the topography of the underlying structures. Besides the significance to technological applications, our experiments pose some important questions regarding the structure of stationary probability distributions in non-equilibrium systems. Colloidal particles undergo perpetual Brownian motion resulting from the stochastic and rapid collisions with solvent molecules. As a result, an ensemble of colloidal particles spreads diffusively to fill all available space and maximize configurational entropy. Restriction of particles to a specified region requires work of an external field that makes target configurations energetically favourable. Boltzmann’s distribution, in fact, predicts that the resulting stationary density of non-interacting particles is a local function of energy alone, whatever is the path that a particle must trace to reach that point. On the other hand, active particles, like swimming bacteria or chemically propelled colloids, are animated by a non-equilibrium stochastic force that is usually characterized by a persistence time on the timescale of seconds [1] , [2] , [3] . When the persistence length of the resulting trajectory is large enough to probe asymmetric features in rigid obstacles, the flux of active particles can be efficiently rectified. Galajda et al. [4] have shown that bacteria concentrate in one-half of a bipartite chamber, when the separating wall is made of asymmetric, funnel-shaped apertures. When the asymmetric wall is actually the outer boundary of a mobile object, bacteria can also self-organize around it and give rise to a net rotary motion [5] , [6] . Random walks, with a finite persistence length, are also observed in passive colloidal tracers, which are suspended in a bath of swimming bacteria [7] , [8] , [9] . The resulting off-equilibrium dynamics can give rise to novel phenomenology, as, for example, the appearance of short-range effective attractions between otherwise repulsive colloids [10] . It is then natural to ask whether it is possible to rectify also these random walks to deliver passive colloidal cargoes to target locations. This would have a clear technological relevance for the design of autonomous microdevices that could be able to collect and sort non-motile bodies in a predictable way. In previous attempts to use bacteria for colloidal delivery, motile cells have been attached on the cargo surface and used as tiny micro propellers [11] , [12] , [13] , [14] . However, external stimuli are required to steer the propellers and trigger cargo release [15] , [16] , [17] , [12] , [18] . The resulting delivery is quite fast but requires a constant external feedback to work. Here we demonstrate that it is possible to design 3D structures such that passive colloids can be spatially organized by a suspension of swimming bacteria. Bacteria can spontaneously deliver an initially homogeneous ensemble of 2 μm colloids into a 16 × 16 μm 2 accumulation area within a timescale of 20 min. The mechanism does not require any attachment of bacterial propellers to colloidal cargoes nor any external control fields. It rather rectifies the off-equilibrium fluctuating forces that arise from the bacterial bath to obtain the required work. Basic principle and experimental implementation The basic principle in our method is illustrated in Fig. 1a . Let us suppose we have an ensemble of non-interacting Brownian particles hopping between two metastable states 0 and 1 that have the same energy and the same spatial extent δ . For an equilibrium thermal bath, the number n 0 of particles in the state 0 is equal to n 1 independently of the energy barrier shape. However, the situation may dramatically change in the presence of a noise fluctuating with a finite correlation time. In the limiting case of a force persistence time that is much larger than transition time, then the probability of jumping from 0 to 1 is related to the probability of being pushed by the bath with a force of amplitude ξ larger than the slope of the energy barrier f 0 . As, in general, a large ξ will be less frequent than a small ξ , transitions from 1 to 0, that involve climbing over a smaller slope, will be more frequent than the reverse transitions from 0 to 1. The resulting imbalance in the transition rates will lead to a stationary state where the bead spends more time in 0 than in 1. In particular, the stationarity condition n 0 λ 01 = n 1 λ 10 will give n 0 =( λ 10 / λ 01 ) n 1 where λ 01 is the rate of transition from 0 to 1, whereas λ 10 is the rate of the reverse transitions. Such simple reasoning can be readily extended to the more complex case where a two-dimensional region 0 is surrounded by multiple asymmetric walls defining a series of connected regions 0,1,2,… as in Fig. 1b . In the case where , the number of particles in the inner region can be amplified by a factor ( λ + / λ − ) m , where m is the number of barriers. If the transition rates are unbalanced by a factor 2, then three walls are enough to achieve an order of magnitude change in particle density. We have implemented asymmetric energy barriers by patterning a flat surface with a 3D structure. The gravitational forces acting on sedimenting beads translate the topography of the surface into an energy landscape. We then use motile bacteria to drive colloidal beads with off-equilibrium stochastic forces with a finite persistence time ( Fig. 1c ). 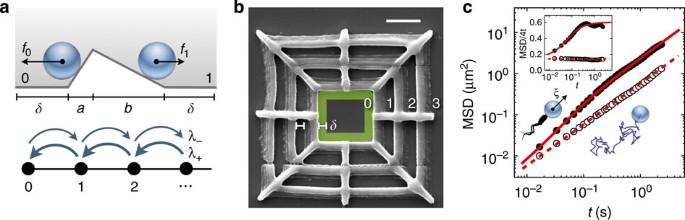Figure 1: Basic principle and experimental conditions. (a) A schematic representation of the main geometric and dynamic features of transitions between states separated by asymmetric barriers. (b) A scanning electron microscopy image of a square structure that gathers particles to the centre. Radial walls provide an increased structural stability. Scale bar, 10 μm in length. (c) The mean squared displacements (MSD) of the beads in the absence of bacteria (simple Brownian motion, open symbols) and in the bacterial bath (filled symbols). Solid and dashed lines are fits to the data (see Methods) giving a persistence time ofτc=0.04 s for the active system. Inset depicts the same data as an effective diffusivity (divided by 4τ), clearly showing the super diffusive regime at short times. We extract a simple Brownian diffusivity ofD0=0.15 μm2s−1, whereas after adding bacteria we observe an additional active termDA=0.45 μm2s−1. Figure 1: Basic principle and experimental conditions. ( a ) A schematic representation of the main geometric and dynamic features of transitions between states separated by asymmetric barriers. ( b ) A scanning electron microscopy image of a square structure that gathers particles to the centre. Radial walls provide an increased structural stability. Scale bar, 10 μm in length. ( c ) The mean squared displacements (MSD) of the beads in the absence of bacteria (simple Brownian motion, open symbols) and in the bacterial bath (filled symbols). Solid and dashed lines are fits to the data (see Methods) giving a persistence time of τ c =0.04 s for the active system. Inset depicts the same data as an effective diffusivity (divided by 4 τ ), clearly showing the super diffusive regime at short times. We extract a simple Brownian diffusivity of D 0 =0.15 μm 2 s −1 , whereas after adding bacteria we observe an additional active term D A =0.45 μm 2 s −1 . Full size image Our structures were built using a diffractive maskless lithography technique, utilizing coherent laser light focused through a microscope objective and shaped by a spatial light modulator with computer-generated holograms. Thus, high-intensity laser spots can be projected onto a photopolymer allowing for micron-featured polymerization [19] . Figure 1b shows a scanning electron microscopy image of a device composed by a series of three square boundaries having the larger slope pointing towards the inner region. Structures of this kind are designed to collect particles in the innermost chamber. By simply reversing the direction of the slopes, we can build devices that are expected to eject beads outside. Supplementary Fig. S1 provides a tilted scanning electron microscopy image as well as 3D reconstructions of collecting and ejecting structures. The final structures approximately have a vertical height of 2 μm, with slopes shaped by horizontal distances of a =0.5 μm and b =2 μm ( Fig. 1a ). The thermal sedimentation length for our colloidal particles is 0.1 μm corresponding to an energy barrier of 20 k B T . As a consequence, in the absence of bacteria, particles are strictly confined by the walls. On the other hand bacteria are expected to have a much higher effective sedimentation length because of both their lower buoyancy mass and higher diffusion constant. As a consequence, the structures only provide a shallow landscape for bacteria that are expected to easily swim above them and to show no tendency to accumulate or deplete in their interior. Observation of colloidal accumulation and depletion by bacteria In Fig. 2a , we digitally track colloidal beads, shown in green, on a surface with collecting and ejecting structures. Initially, after all beads are sedimented, we have a surface number density that, by direct counting, we find to be ρ c =0.013 μm −2 . We set time t =0 soon after the introduction of bacteria, while the distribution of beads is still homogeneous and the concentration of cells is uniform. For the same experiment, the surface number density of bacteria is ρ b =0.014 μm −2 . After about 20 min, the collecting structures are filled up, while ejecting structures have expelled all colloidal beads ( Fig. 2b ). A time-averaged histogram of bead positions during the last 5 min of the run ( Fig. 2c ) shows marked accumulation and depletion. In the absence of bacteria, however, the particles, driven solely by thermal fluctuations, remain trapped in the structures’ compartments ( Fig. 2d ). Boltzmann statistics would predict a uniform probability density throughout the flat regions in our system all corresponding to the same energy level. A colloidal density of ρ c =0.013 μm −2 corresponds to an average of 3.3 particles in the inner regions of the collecting structures. In the absence of bacteria, collecting structures at the top left and bottom right of Fig. 2d contain, respectively, two and seven particles. Assuming a Poisson probability distribution, those configurations are expected to occur with corresponding probabilities of 20 and 3%. On the contrary, after the addition of bacteria, the same two structures contain an average of 13 particles over the last 40 s ( Fig. 3 ). That would only occur with a probability 0.003% assuming again a uniform probability distribution as in equilibrium. 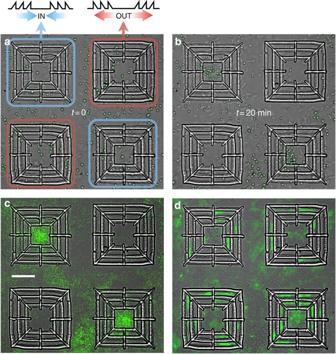Figure 2: Observation of particle concentration and depletion by bacteria. Single experiment snapshots of particles and bacteria at the initial statet=0 where particles are randomly distributed (a) and fort=20 min, where particle distributions have been strongly affected by bacterial transport over asymmetric barriers (b). We highlight in green the colloidal particles that are not stuck on the surface. Particle distributions averaged over a steady state are shown incfor particles in the bacterial bath betweent1=15 min andt2=20 min (Δt=5 min) and indfor particles in an experiment without bacteria, undergoing simple Brownian motion for Δt=10 min. In the absence of bacteria, the colloidal particles remain trapped within the structures compartments. Scale bar, (c) 20 μm. Figure 2: Observation of particle concentration and depletion by bacteria. Single experiment snapshots of particles and bacteria at the initial state t =0 where particles are randomly distributed ( a ) and for t =20 min, where particle distributions have been strongly affected by bacterial transport over asymmetric barriers ( b ). We highlight in green the colloidal particles that are not stuck on the surface. Particle distributions averaged over a steady state are shown in c for particles in the bacterial bath between t 1 =15 min and t 2 =20 min (Δ t =5 min) and in d for particles in an experiment without bacteria, undergoing simple Brownian motion for Δ t =10 min. In the absence of bacteria, the colloidal particles remain trapped within the structures compartments. Scale bar, ( c ) 20 μm. 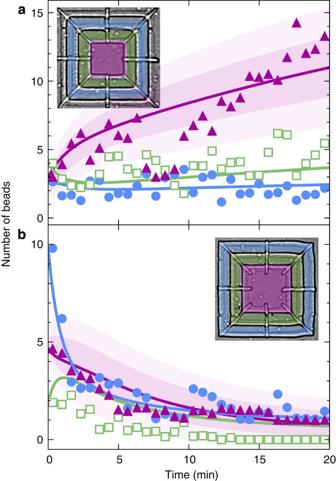Figure 3: Temporal evolution of particle numbers within structural compartments. Particle numbers from a single experiment are averaged between the two collecting (a) and ejecting (b) structures shown inFig. 2. Each structure is divided into three compartments as highlighted by shaded areas in the insets: centre (purple, triangles), middle (green, squares) and outer (blue, circles). Solid lines represent the best fit solution to the rate equation model described in the text. Shaded areas in the plot represent the expected one and two s.d. limits for predicted fluctuations in the evolution of beads numbers. Full size image Figure 3: Temporal evolution of particle numbers within structural compartments. Particle numbers from a single experiment are averaged between the two collecting ( a ) and ejecting ( b ) structures shown in Fig. 2 . Each structure is divided into three compartments as highlighted by shaded areas in the insets: centre (purple, triangles), middle (green, squares) and outer (blue, circles). Solid lines represent the best fit solution to the rate equation model described in the text. Shaded areas in the plot represent the expected one and two s.d. limits for predicted fluctuations in the evolution of beads numbers. Full size image Temporal evolution and transition rate modelling To get a quantitative estimate of the transition rates, we have recorded the time evolution of the number of beads in the three internal regions of all structures. Averaged data, corresponding to the two collecting and ejecting structures in Fig. 2 , are reported in Fig. 3 . As a starting model, we assume that the number of beads in each region is governed by a coupled set of linear rate equations. Calling N =( n 0 , n 1 , n 2 ) the array of particle numbers we have: with Λ the rate matrix: and S =(0,0, s ) a source term, where s is the probability per unit time that a bead enters the structures from the outside. As in the states 1 and 2, the beads are confined to be within the same distance δ from the two walls, it is reasonable to assume that λ 12 = λ 23 = λ out and λ 21 = λ 10 = λ in . However, we can expect that λ 01 is significantly lower than λ 12 as beads in 0 are on average at a larger distance from the wall. We correct for this effect by assuming λ 01 = αλ out , with α <1 being the probability for a bead in region 0 to be located within a distance from the wall equal to δ . We estimate α as the ratio between the shaded area in Fig. 1c and the total area of region 0. With reference to Fig. 1a , the values of λ in and λ out will correspond, respectively, to λ + and λ − for the collecting structures and to λ − and λ + for the ejecting ones. The formal solution of equation (1) reads: with the stationary state N (∞)= Λ −1 S . Defining as the constant average number of beads that lay within a distance δ from the outer wall, we can write s = λ in and have n 0 (∞)=α( λ in / λ out ) 3 . This model completely neglects the excluded volume interactions between particles, which will set a maximum number of beads that a structure can accommodate in its interior. Nevertheless, we find a single set of fitting parameters λ + , λ − and that describes well the observed filling and emptying processes on both the structures ( Fig. 3 ). In particular, we obtain λ + =0.66 min −1 and λ − =0.36 min −1 with a ratio λ + / λ − of ~2. The fitted value of is 1.8, which is of the order of the average number of particles laying within a distance δ from the outer boundary of the structure. The fitted curves are reported as solid lines in Fig. 3 . In addition, for the innermost regions, we also report as shaded areas the expected one and two s.d. limits for fluctuations. Although data for ejecting structures seem to show a reasonable noise level, the number of particles in the centre of collecting structures shows extremely large fluctuations. We believe that those fluctuations may arise from collective effects that are neglected in our simple analysis but are likely to be important once colloidal beads start to pack together. However, there are systematic and reproducible accumulation effects across multiple and independent experiments as shown in Fig. 5 . 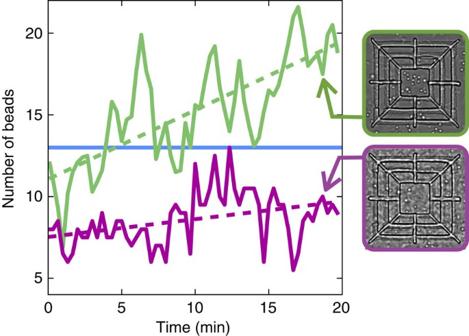Figure 4: Effect of bacterial density on filling efficiency. Solid lines represent the time evolution of total beads count over entire filling structures in the case of low- and high-bacteria densities:ρb=0.014 (green) and 0.2 (purple) μm−2. The constant blue line shows the unchanging particle number in the absence of bacteria. Figure 4: Effect of bacterial density on filling efficiency. Solid lines represent the time evolution of total beads count over entire filling structures in the case of low- and high-bacteria densities: ρ b =0.014 (green) and 0.2 (purple) μm −2 . The constant blue line shows the unchanging particle number in the absence of bacteria. 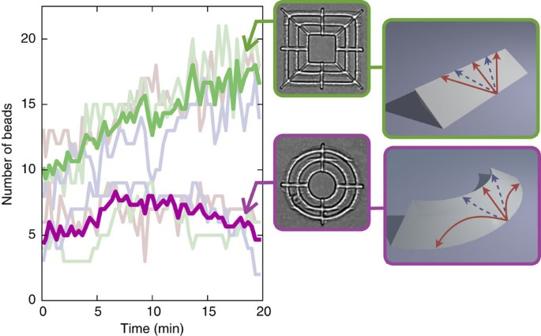Figure 5: Filling efficiency for collecting structures of different curvatures. Thick solid lines represent a bead number average over three different experiments on the total surface of nearby square (green) and circular (purple) structures. Unaveraged curves are displayed in the background and colour coded to each iteration. In addition, we show a schematic of the effect of wall curvature on the trajectory of a particle driven by constant propelling force. Dotted arrows show the trajectories without gravity. In the presence of gravity, the flat ramp applies a constant force, whereas the curved ramp results in a position-dependent force, which is able to deflect particles more easily. Full size image Figure 5: Filling efficiency for collecting structures of different curvatures. Thick solid lines represent a bead number average over three different experiments on the total surface of nearby square (green) and circular (purple) structures. Unaveraged curves are displayed in the background and colour coded to each iteration. In addition, we show a schematic of the effect of wall curvature on the trajectory of a particle driven by constant propelling force. Dotted arrows show the trajectories without gravity. In the presence of gravity, the flat ramp applies a constant force, whereas the curved ramp results in a position-dependent force, which is able to deflect particles more easily. Full size image Role of bacterial concentration It is expected that the jump rates and steady-state probabilities will depend on many parameters, the simplest of which are the height and slopes of the structures. Other parameters include particle size and density or the bacterial concentration and motility. In particular, we find that when the bacterial density is increased, beads acquire a higher diffusivity that makes them less sensitive to the action of the underlying landscape. In Fig. 4 , we report time evolution of the number of beads over an entire collecting structure for the three cases ρ b = 0, 0.014 and 0.2 μm −2 . As expected, an increased activity leads to a balancing of the two rates λ + and λ − with the consequent weakening of rectification. We do not observe any appreciable accumulation effects for swimming bacteria since diffusivities, in that case, are extremely large. Structural curvature effect A rather unexpected and significant result appears by modifying the curvature of the structures from square boundaries to circular ones ( Fig. 5 ). Although both barriers have the same profile, square structures are much more effective in collecting particles than circular ones. We hypothesize that the effect of curvature is connected to the narrowing of incident angles for which a bead, driven by a constant force, is allowed to surpass the barriers. Currently although, we cannot exclude the possibility of contributions to this effect from modification of the noise near the boundaries because of complex bacteria-particle–wall interactions. We have conceived and implemented a novel method to use self-propelled bacteria as micro propellers that are capable to transport and segregate colloids over micro-patterned structures. The proposed mechanism relies on the use of bacteria as the source of an off-equilibrium noise that allows colloidal particles to cross asymmetric barriers with strongly biased transition rates in opposite directions. The fact that the combination of an asymmetric energy landscape and an off-equilibrium-coloured noise leads to the appearance of non-zero fluxes is a well-known result of statistical mechanics [20] , [21] , [22] . However, the relevance and the potentiality of this kind of rectification process for self-propelled particles has been recognized only very recently and mostly in theoretical and idealized situations [3] , [23] . Previously reported rectification phenomena in active matter rely on a different effect where the presence of geometric constraints drives self-propelled particles along non-reversible paths [4] , [24] . In contrast, here active particles are free from strict geometric constraints and rectification arises from asymmetries in the field of applied forces. As opposed to the case of two-dimensional funnel-shaped obstacles, that only provide a limited number of rectifying channels, our asymmetric 3D barriers can be crossed with biased rates at any point along their length, allowing for an increased rectification efficiency. Moreover, we use bacteria to segregate passive heavy colloidal particles, whereas the active bacterial component is basically unaffected by the underlying structure. It is also important to note that, as the rectification process here is driven by transitions over energy barriers that are well above k B T , the disruptive effects of Brownian motion to rectification are significantly reduced. Further investigations on the role of barrier shape could lead to the design of optimal devices having a higher and faster collection efficiency and that could discriminate between colloids of different size, shape or density. Microfabrication Microfabrication is performed through a holographic optical tweezer set-up [25] , [26] with a reflective liquid crystal SLM (Holoeye LC-2500) to impose a computer-generated pattern of phase shifts [27] generated by NVIDIA CUDA parallel processing [28] on an expanded laser beam (Diode Pumped Solid State (DPSS) Opus Ventus 532 nm, 3 W). The emerging wavefront is focused by a large numerical aperture microscope objective (Nikon Plan Apo VC 100 × , numerical aperture 1.4) onto an array of spots as determined by the parameters of the structure being built. As a patterning photopolymer, we used Norland NOA 63, an ultraviolet curing adhesive. Although, the adhesive sensitivity lies outside the wavelength of the laser, the low absorption allows for intensity-based threshold processing [19] . After fabrication, the uncrosslinked glue was removed by gently washing with toluene and then drying in open air. Cell growth Escherichia coli cells (MG1655) were grown overnight at 33 °C in tryptone broth (Fluka) containing 1% tryptone. The saturated culture was then diluted 1:100 into fresh medium and grown for 4.5 h at 33 °C and mildly shaken at 200 r.p.m. Bacterial cells were then collected from culture media by centrifugation at 2,000 r.p.m. for 10 min at room temperature. The resulting pellet was gently resuspended by mixing in pre-warmed motility buffer (10 −2 M glucose C 6 H 12 O 6 , 10 −4 M EDTA (pH 7.0) and 0.2 % Tween 20) [29] . This process was repeated in total three times for replacing the growth medium with motility buffer and halt bacterial growth. No salts were added to the growth medium or the motility buffer to avoid particle aggregation and adhesion to the cover glass. We have observed no significant change in the growth and motility characteristics of our bacteria in these salt-free media. Sample preparation A surfactant solution of 1% Tween 20 was applied on the glass coverslips, let to dry and placed in a microscope coverslip holder. Silica beads of 2 μm diameter (Bangs Laboratories Inc.) were dispersed in the bacterial motility buffer. Colloidal solution (2.5 μl) was added to the coverslip surface, followed by a 2.5 μl of bacterial solution, resulting in a sample height of the order of 150 μm. The holder was then sealed and humidity throughout the experiment was maintained with a damp cloth. Particle imaging Images were acquired with × 20 and × 40 Nikon Plan Fluor objectives in a bright-field microscopy set-up. Particle tracking was accomplished through a centre of mass algorithm after subtracting the average background and applying a threshold. Particle numbers in structures were initially taken from tracking and then verified by observation and counting. To extract the persistence time and diffusivities, the two-dimensional mean-squared displacements were fitted by a simplified active diffusion model [7] with an extra short-time Brownian diffusive term: with τ c the correlation time, D A the long-time active diffusivity and D 0 the Brownian diffusivity. How to cite this article: Koumakis, N. et al. Targeted delivery of colloids by swimming bacteria. Nat. Commun. 4:2588 doi: 10.1038/ncomms3588 (2013).